On-chip transformation optics for multimode waveguide bends Current optical communication systems rely almost exclusively on multimode fibres for short- and medium-haul transmissions, and are now expanding into the long-haul arena. Ultra-high bandwidth applications are the main drive for this expansion, based on the ability to spatially multiplex data channels in multimode systems. Integrated photonics, on the other hand, although largely responsible for today’s telecommunications, continues to operate almost strictly in the single-mode regime. This is because multimode waveguides cannot be compactly routed on-chip without significant inter-mode coupling, which impairs their data rate and prevents the use of modal multiplexing. Here we propose a platform for on-chip multimode devices with minimal inter-mode coupling, opening up the possibilities for integrated multimode optics. Our work combines a novel theoretical approach—large-scale inverse design of transformation optics to maximize performance within fabrication constraints—with unique grayscale-lithography fabrication of an exemplary device: a low-crosstalk multimode waveguide bend. In principle, inter-modal mixing does not occur for multimode propagation in a perfectly straight waveguide, but when bends (or other perturbations to the guiding structure) are introduced, mixing between the modes can be significant. Any deviation from the straight path of the waveguide will cause excitation of many other modes, because of the modal mismatch between the straight and curved sections. The modal superposition thus created would limit the data rate that this waveguide can support [1] . We demonstrate here signal routing in a multimode waveguide bend with ultra-low inter-mode coupling designed using transformation optics (TO) [2] , [3] . The design is based on the curving of a virtual space containing the straight multimode waveguide into a 90° bend, such that light travels along the curve as it would on the original straight waveguide, that is, with minimal inter-mode coupling. It is important to observe that not only is the modal distribution preserved throughout the bend but also is the phase relationship between modes, a key factor for any phase-sensitive application. Modal crosstalk in multimode waveguides The modal superposition excited in multimode bends is exemplified in Fig. 1 , where we show the field distribution of a 4-μm wide waveguide (supporting 16 modes) excited by the fundamental mode at λ =1.55 μm and bent with 78.8 μm radius. One can see that the bending of the waveguide leads to a superposition of many higher modes at the output, which in turn introduce penalties to the bandwidth of this channel. In the 4-μm waveguide shown in Fig. 1 , the limit in bandwidth-distance product that can be supported only due to difference in group velocities between the fundamental and second-order mode is below 16 Gb m s −1 (for complete symbol overlap), between the fundamental and third-order mode is 6 Gb m s −1 , and so on. Therefore, any device that couples a significant amount of power into these modes, such as the circular bend simulated here (71% of the power input in the fundamental mode is coupled to the second-order mode and 23% to the third), will severely limit the communication data rate of the system. One way to minimize the mode mixing would be to use very large bending radii. For the 4-μm waveguide, to ensure that 95% of power is coupled back to the fundamental mode of the straight waveguide, a bending radius of more than 1 mm is necessary, which is unacceptably large for photonics integration. 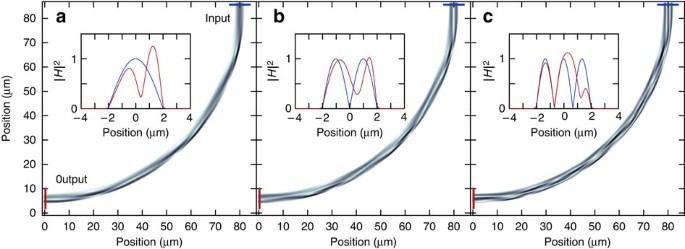Figure 1: Finite element simulations of a multimode bend. The figure shows the magnetic field magnitude squared (|H|2) for a conventional multimode bend when excited with the first three modes of the input multimode waveguide (a–c, respectively). The input modes (blue cross-sections, on the upper-right endpoints) are coupled to many other modes, as evidenced by the cross-section plots at the outputs (red, on the lower left endpoints). The waveguides are 4 μm wide and the bends have 78.8 μm radius. The simulations were performed using the FEniCS solver4. Figure 1: Finite element simulations of a multimode bend. The figure shows the magnetic field magnitude squared (| H | 2 ) for a conventional multimode bend when excited with the first three modes of the input multimode waveguide ( a – c , respectively). The input modes (blue cross-sections, on the upper-right endpoints) are coupled to many other modes, as evidenced by the cross-section plots at the outputs (red, on the lower left endpoints). The waveguides are 4 μm wide and the bends have 78.8 μm radius. The simulations were performed using the FEniCS solver [4] . Full size image Multimode bend design via TO There are two main challenges in designing a waveguide bend via TO in a silicon photonics platform, in contrast to arbitrary metamaterials [5] , [6] , [7] , [8] . The first design challenge is the need to employ only isotropic materials with refractive indices limited to values between the index of Si and the index of SiO 2 (roughly 1.5< n <3.5). Although in principle anisotropic materials, such as SiC, can be used in silicon photonics, TO requires in general a gradient anisotropy, which is much more complex to achieve. Note that one could also use photonic crystals [9] , [10] , [11] , [12] or grooves [13] , [14] to tailor the index and anisotropy, however these discrete structures result in additional field scattering and inter-mode coupling due to the finite wavelength/period ratio (typically around 10:1). Instead, we use a grayscale-lithography technique described below that produces smooth gradients but is limited to mostly isotropic effective indices. The second design challenge is to match the refractive index and the geometry of the device at its endfacets to the multimode waveguides connected to it. If the connection is not matched, each mode from the straight waveguide will couple to many modes in the bend, similar to the case of a conventional bend ( Fig. 1 ), immediately introducing inter-mode coupling, even if the bend itself does not. This means that the bend transformation must smoothly transition from the same shape of the input waveguides at its endfacets to the required curve in its interior. To address these two design challenges, we developed a general optimization method for TO design of the profile and dimensions of the multimode devices for minimal inter-modal mixing, while accounting for limited index contrast and anisotropy, and at the same time ensuring minimal reflections at the interfaces. We optimize the design of the structure over a large space of possible smooth transformations, parameterized by general Fourier/Chebyshev series coefficients, to find the transformation with minimal worst-point anisotropy that satisfies the refractive index constraints (see Methods). At the same time, we match the geometry and index of the bend endfacets to the adjacent multimode waveguide—the transformation is parameterized in such a way as to satisfy this boundary condition by construction. Note that previous quasi-conformal maps proposed to minimize transformation anisotropy [15] , do not incorporate the index constraints, minimize only the average anisotropy and require the entire boundary curves of the bend shape to be specified a priori instead of just the endfacet locations. The optimized multimode bend obtained has an effective radius of curvature of 19.7 times the width of the waveguide. Using a 4-μm wide waveguide then results in a radius of 78.8 μm, which we also used in the simulations of Fig. 1 for comparison. In Fig. 2 , we show the first three propagating modes of the input waveguide travelling almost undisturbed through the optimized bend. The optimized bend's effective-index profile can be seen in Fig. 3a . 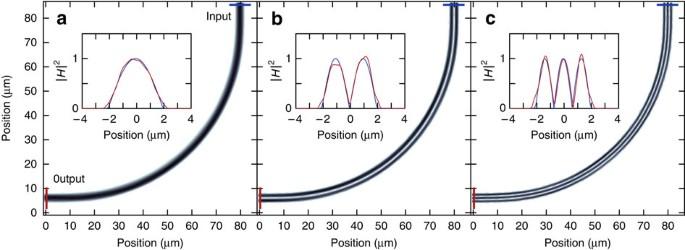Figure 2: Finite element simulations of our optimized TO multimode multimode bend. The figure shows the magnetic field magnitude squared (|H|2) for the cases when the bend is excited with the first three modes of the input multimode waveguide (a–c, respectively). The input modes (blue cross-sections, on the upper-right endpoints) are preserved throughout the bends, showing minimal inter-mode coupling at the outputs (red, on the lower left endpoints). The waveguides are 4 μm wide and the bends have 78.8 μm radius. Figure 2: Finite element simulations of our optimized TO multimode multimode bend. The figure shows the magnetic field magnitude squared (| H | 2 ) for the cases when the bend is excited with the first three modes of the input multimode waveguide ( a – c , respectively). The input modes (blue cross-sections, on the upper-right endpoints) are preserved throughout the bends, showing minimal inter-mode coupling at the outputs (red, on the lower left endpoints). The waveguides are 4 μm wide and the bends have 78.8 μm radius. 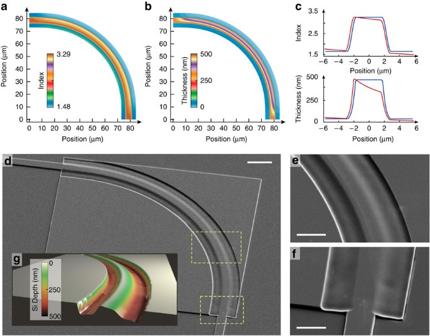Figure 3: TO design and fabrication. Optimized refractive index profile (a) for the multimode bend and respective silicon layer thickness (b) to implement the bend. (c) Cross-sections of the refractive index and thickness of the profiles at the endpoints (blue) and at the centre of the bend (red). (d) Scanning electron microscope images of the fabricated graded-index bend (10 μm scale). The smoothness obtained by our grayscale process can be seen in panele, the close-ups of the bend interior (5 μm scale), and panelf, the connection with a conventional multimode waveguide at the output (4 μm scale). (g) Atomic force microscope scan of a fabricated bend, showing the thickness profile in the silicon layer. Full size image Figure 3: TO design and fabrication. Optimized refractive index profile ( a ) for the multimode bend and respective silicon layer thickness ( b ) to implement the bend. ( c ) Cross-sections of the refractive index and thickness of the profiles at the endpoints (blue) and at the centre of the bend (red). ( d ) Scanning electron microscope images of the fabricated graded-index bend (10 μm scale). The smoothness obtained by our grayscale process can be seen in panel e , the close-ups of the bend interior (5 μm scale), and panel f , the connection with a conventional multimode waveguide at the output (4 μm scale). ( g ) Atomic force microscope scan of a fabricated bend, showing the thickness profile in the silicon layer. Full size image Graded-index device fabrication The fabrication of this multimode bend is achieved using grayscale e-beam lithography, on a silicon-on-insulator wafer with 3 μm buried SiO 2 and 500 nm Si layer. We create the required non-uniform refractive index medium using the effective propagation index for our vertical slab structure, composed by the buried SiO 2 layer, the guiding Si layer and a cladding layer of SiO 2 deposited via plasma-enhanced chemical vapour deposition. The effective propagation index of this structure is controlled by the thickness of the Si layer [16] , [17] , [18] , [19] , [20] , such that the index map from the TO optimization ( Fig. 3a ) is translated into a thickness map to be fabricated via grayscale lithography ( Fig. 3b ). The grayscale lithography is achieved via dose modulation for patterning the photonic device with vertical resolution of ~10 nm. Note that although similar processes are employed in the fabrication of diffractive optical elements, micro-electro-mechanical structures and lower contrast graded-index lenses [21] , [22] , [23] , [24] , [25] with relatively weak height variations of 80 nm over distances of tens of microns, in our case, the process enables strong height variations of 400 nm over less than 1 μm while maintaining precise control of both the resist height profile on the nanometre scale. Figure 3 shows the grayscale patterned device with a smooth surface profile in Si. To evaluate the performance of our mode-preserving multimode bend, we compare it with a circular multimode bend with rectangular profile and with same radius as our device (78.8 μm). We measure the transmission coefficient of the fundamental mode through the bend, so that the presence of inter-mode coupling is evidenced by low transmitted power in the system. To ensure we are exciting and collecting only the fundamental waveguide mode, we couple light into our sample via a grating connected to a single-mode waveguide, which, in turn, tapers very slowly (over 250 μm) to a 4-μm wide multimode waveguide. This waveguide connects to the bend and the output is once again slowly tapered down to a single-mode waveguide, radiating away any higher-order modes that might have been excited along the bend. Light from the single-mode waveguide is coupled via another grating to a fibre, which in turn is connected to detector and a power meter. An optical microscope image of this system is shown in Fig. 4a . The results are displayed in the plots of Fig. 4b , where we show the histograms for measurements of 25 devices designed via TO and 11 conventional multimode bends. 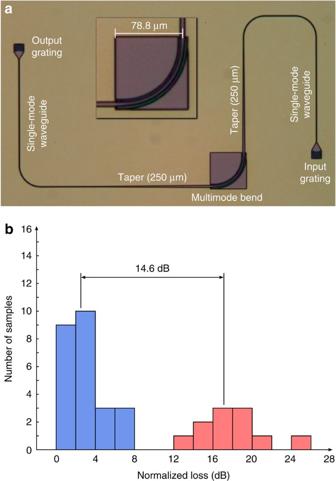Figure 4: Multimode bend experiment. (a) Optical microscope image of a tested device. Because of the large length of the tapers, only the fundamental mode is excited at the multimode bend input. Conversely, higher-order modes excited along the bend are radiated by the output taper, such that the power measured at the output grating reflects how well the fundamental mode is preserved by the bend. (b) Histograms of the measurements from our multimode bend design (blue) and a conventional multimode bend with rectangular cross-section (red) with same radius. There is a 14.6-dB improvement in the average transmission coefficient for the fundamental mode of the optimized bend with respect to the conventional one. Figure 4: Multimode bend experiment. ( a ) Optical microscope image of a tested device. Because of the large length of the tapers, only the fundamental mode is excited at the multimode bend input. Conversely, higher-order modes excited along the bend are radiated by the output taper, such that the power measured at the output grating reflects how well the fundamental mode is preserved by the bend. ( b ) Histograms of the measurements from our multimode bend design (blue) and a conventional multimode bend with rectangular cross-section (red) with same radius. There is a 14.6-dB improvement in the average transmission coefficient for the fundamental mode of the optimized bend with respect to the conventional one. Full size image The data presented in Fig. 4b clearly show the vast improvement in transmission from our TO multimode bends with respect to the conventional ones, a direct result of the mode-preserving characteristic of our design. Moreover, the two-dimensional (2D) simulations in Figs 1 and 2 show a difference in transmission for the fundamental mode of 13.6 dB, closely agreeing with the experimental results. It is also important to analyse the performance of our multimode bend against a conventional single-mode one to evaluate how much the grayscale fabrication impacts in the total losses in the link. Measurements of 11 single-mode waveguide bends on the same sample showed an averaged normalized transmission coefficient of −2.6 dB, very similar to our TO design (−2.5 dB). These numbers enforce our conclusions of minimal inter-mode coupling in the optimized bend and indicate that any additional losses introduced in the grayscale process are compensated by the naturally lower losses found in multimode waveguides (due to less interaction of the fields with the core interfaces). We note that the variations in the transmission seen in the measurements of the TO bend are observed in the single-mode devices as well, indicating that the variations are due to fabrication steps common to all devices, which might have introduced impurities in the sample, and not from the grayscale process itself. Thus, we demonstrate an optimized design and fabrication process for a multimode photonic platform with very low inter-mode coupling. This platform can be used to enable multimode photonics while also pointing towards the possibility of developments in mode multiplexing [26] , [27] , [28] , [29] , [30] for ultra-high bandwidth communications. Optimization details The idea of TO [3] , [31] is that the effects of coordinate transformations with Jacobian in 2D can be converted into a choice of materials. In the special case that the original material (relative permittivity ε = n 2 , relative permeability μ =1) is isotropic and non-magnetic, the material indices become where n ( x , y ) is the index profile of the untransformed structure. Furthermore, if ε ′ and μ ′ are slowly varying compared with the wavelength, then μ ′ can be approximately commuted with the × in Maxwell's equations and combined with ε ′ to yield an effective dielectric-only index of refraction tensor [15] It is desirable to choose a transformation that minimizes the anisotropy. One possible measure of this anisotropy is the function [15] : where and are the square roots of the two eigenvalues of . Ref. 32 called the “Liao functional”, which measures an average anisotropy, and refs 15 , 33 noted that it is minimized by ‘quasi-conformal maps’. A low-anisotropy transformation is then approximated by an isotropic root mean square index Although ref. 15 suggested that minimizing the mean anisotropy would also minimize the maximum anisotropy, we found that minimizing the average anisotropy in some circumstances could still yield large localized anisotropy spikes (which cause scattering in the approximate isotropic structure), so we instead minimize the maximum of . Our bend transformation can be decomposed into two steps, as shown in Fig. 5 . First, the rectangular segment of length L ( x , y [0,1] × [− L /2,+ L /2]) is transformed into a circular bend of radius R with the polar coordinates r = R + x and θ = πy /(2 L ). This simple bend is highly anisotropic, so in the second step, we introduce arbitrary additional perturbations δ r and δ θ (not necessarily small) into this transformation, obtaining and . The final transformation is then and . We minimize the maximum anisotropy max over a large space of these perturbation functions and . 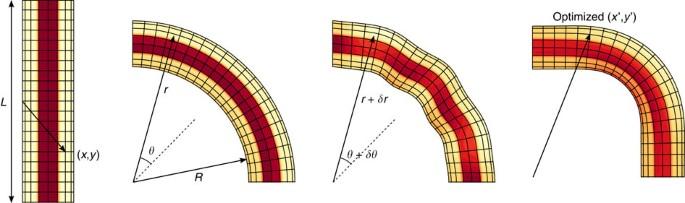Figure 5: Schematic of three-step bend transformation. We start with a mapping of a straight region of lengthLto a stretched circular bend of radiusR, and then further perturb the coordinates. After the perturbation, we compute the anisotropy and index of refraction (darker areas have higher index). Finally, we optimize the original lengthLand coordinate perturbations δrand δθfor minimum anisotropy. With these definitions, the trace and determinant in the expressions for and n take the simple form Figure 5: Schematic of three-step bend transformation. We start with a mapping of a straight region of length L to a stretched circular bend of radius R , and then further perturb the coordinates. After the perturbation, we compute the anisotropy and index of refraction (darker areas have higher index). Finally, we optimize the original length L and coordinate perturbations δ r and δ θ for minimum anisotropy. Full size image As we are interested only in smooth transformations, we parametrize δ r and δ θ in a spectral basis [34] : by the coefficients of Chebyshev polynomials T l in the x (radial) direction and Fourier series in the y (angular) direction. The reason δ r only has cosine terms and δ θ only has sine terms is that we restrict ourselves to bends that are mirror symmetric about the midline ( θ =0). The factor of 1/( R + x ) has been inserted for convenience in satisfying a continuity boundary condition discussed below. Because of the exponential convergence of such expansions for smooth functions [34] , we found it sufficient to use l =0…5 and m =0…7 to obtain convergence. There are several boundary conditions that we must consider. First, the ends of the bend must couple smoothly into straight waveguides. Hence, δ r =δ θ =0 at the ends, to coincide with the ends of a circular bend. The sine series of δ θ automatically satisfies this. However, the Dirichlet condition on the cosine series of δ r must be manually imposed by evaluating the cosine at the endfacets y =± L /2 for each l in the Chebyshev series: With these boundary conditions, the gradients at the endfacets become and . Hence, the transformed isotropic (root mean square) index at the ends y =± L /2 is For the endfacet to couple directly into the straight waveguide, must coincide with n here. Hence, we must have for all x at the endfacet, which gives the constraint: Finally, there are fabrication constraints: the root mean square index of refraction must lie between 1.45 and 3.2. The bend radius was also chosen to be less than some max value R 0 (otherwise optimization would choose an infinite radius to minimize ). In summary, we formulated the non-linear optimization problem: where G is a grid of sampling points, in our case, a 100 × 300 uniform grid. Here, t is a ‘dummy’ optimization variable introduced to turn the non-differentiable minimax objective (max ) into smooth constraints [35] . In principle, any non-linear-programming algorithm could then be used to find a local optimum of this problem (whereas a global optimum may be much more difficult to find owing to the probable non-convexity). We found it convenient to use the COBYLA algorithm [36] , [37] in the NLopt library [38] . COBYLA is a derivative-free optimization algorithm, which solves a sequence of linear-programming problems formed from linearized approximations of the objective and constraints. At each step, the approximations are constructed via a simplex of d +1 points in d dimensions, and are optimized in a trust region. We found the same (possibly local) optimum was reached for a wide range of starting conditions for the optimization parameters. For example, one possible scheme is to start with all coefficients zero except the last one (to satisfy the coefficient constraints 10, 12). Another scheme is to start with all the coefficients equal. Grayscale lithography The grayscale fabrication process employed was carefully characterized to generate a reproducible dose curve for the e-beam resist, 495K poly(methyl methacrylate) (PMMA), and its etch contrast to Si. The doses used varied from 125 μC cm −2 to about 350 μC cm −2 , resulting in exponentially distributed depths in the PMMA from 20 nm to 360 nm. The resist was developed in a mixture of isopropyl alcohol and deionized water in proportion 2:1 for 1 min. To reduce surface roughness, we reflowed the PMMA for 1 min at 145 °C. Then the sample was etched in an inductively-coupled plasma tool, where the thickness profile patterned on the resist was transferred to the Si layer with a scaling factor determined by the ratio of the etch rates of both materials. How to cite this article: Gabrielli L. H. et al . On-chip transformation optics for multimode waveguide bends. Nat. Commun. 3:1217 doi: 10.1038/ncomms2232 (2012).